Multiple cellular proteins interact with LEDGF/p75 through a conserved unstructured consensus motif Lens epithelium-derived growth factor (LEDGF/p75) is an epigenetic reader and attractive therapeutic target involved in HIV integration and the development of mixed lineage leukaemia (MLL1) fusion-driven leukaemia. Besides HIV integrase and the MLL1-menin complex, LEDGF/p75 interacts with various cellular proteins via its integrase binding domain (IBD). Here we present structural characterization of IBD interactions with transcriptional repressor JPO2 and domesticated transposase PogZ, and show that the PogZ interaction is nearly identical to the interaction of LEDGF/p75 with MLL1. The interaction with the IBD is maintained by an intrinsically disordered IBD-binding motif (IBM) common to all known cellular partners of LEDGF/p75. In addition, based on IBM conservation, we identify and validate IWS1 as a novel LEDGF/p75 interaction partner. Our results also reveal how HIV integrase efficiently displaces cellular binding partners from LEDGF/p75. Finally, the similar binding modes of LEDGF/p75 interaction partners represent a new challenge for the development of selective interaction inhibitors. Lens epithelium-derived growth factor (LEDGF/p75) is an epigenetic reader recognizing H3K36me3 histone marks via its N-terminal PWWP domain [1] , [2] . Knockout of the gene encoding LEDGF/p75 and its splice variant p52 ( Psip1 ) leads to perinatal mortality and severe homeotic skeletal transformations reminiscent of those seen in mice with Hox mutations [3] . LEDGF/p75 has been linked to Hox gene regulation through its interaction with the mixed lineage leukaemia (MLL1)-menin complex [4] . Recent work has revealed that LEDGF/p75 is involved in DNA double-strand break (DSB) repair by the homologous recombination repair pathway, through recruitment of C-terminal binding protein interacting protein (CtIP) to DNA DSB [5] . In addition, LEDGF/p52 has been associated with splicing through its interaction with serine/arginine-rich splicing factor 1 (SRSF1) [1] , [5] . Currently it is not clear whether the previously proposed roles of LEDGF/p75 in apoptosis and stress response, as well as its increased expression levels in different cancer types, are related to one of these functions [6] , [7] , [8] , [9] , [10] , [11] . The Mll gene encodes a histone methyltransferase that forms a ternary complex with LEDGF/p75 and the tumour suppressor menin (MEN1) and is frequently targeted by chromosomal translocations (see ref. 12 for review). Balanced genetic rearrangements result in the formation of new fusion proteins linked to childhood and adult de novo acute leukaemias, as well as therapy-related acute myeloid and lymphoblastic leukaemias. The LEDGF/p75 binding portion of MLL1 is retained in C-terminal fusions (MLL N -fusion), which enables tethering of the MLL N -fusion complexes to MLL1 target genes, resulting in leukaemic transformation. The LEDGF/p75-MLL1-menin complex has been structurally characterized, but the published X-ray data revealed only part of the ternary complex (PDB ID 3U88 (ref. 13 )). Recently, we and others identified a second menin-independent MLL1 binding site on LEDGF/p75 (refs 14 , 15 ). Both interfaces were shown to be important for MLL fusion-mediated transformation and represent valuable novel therapeutic targets [14] , [15] . In addition to its cellular function, LEDGF/p75 has been extensively studied in the context of HIV-1 integration [16] . LEDGF/p75 interacts with HIV integrase (IN) through its C-terminal integrase binding domain (IBD, amino-acid residues 347–429), which is absent in LEDGF/p52 ( Fig. 1 ). This interaction targets viral integration into transcriptionally active regions of the host chromatin recognized by the LEDGF/p75 PWWP domain [17] , [18] , [19] , [20] , [21] . The important role of LEDGF/p75 in lentiviral replication triggered the development of small molecules that efficiently block HIV-1 replication, referred to as LEDGINs that target the LEDGF/p75-HIV IN interaction interface [22] , [23] , [24] , [25] , [26] , [27] , [28] , [29] . LEDGINs are currently under early clinical development. 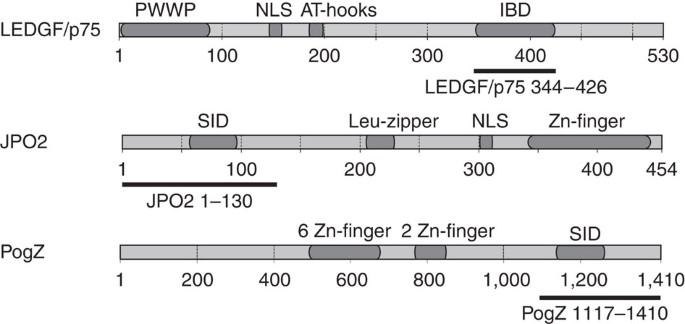Figure 1: Domain organization of LEDGF/p75 and its cellular binding partners JPO2 and PogZ. Regions covered by protein constructs used in this work are represented by black bars. The Pro-Trp-Trp-Pro domain (PWWP), IBD, nuclear localization signal and specific interaction domain are indicated. Figure 1: Domain organization of LEDGF/p75 and its cellular binding partners JPO2 and PogZ. Regions covered by protein constructs used in this work are represented by black bars. The Pro-Trp-Trp-Pro domain (PWWP), IBD, nuclear localization signal and specific interaction domain are indicated. Full size image Since LEDGF/p75 contributes to optimal viral replication and leukaemic transformation and has become a new potential therapeutic target for drug development, it is crucial to study its physiological interactions. In addition to HIV IN and MLL1-menin, the LEDGF/p75 IBD also interacts with CDC7-activator of S-phase kinase complex (CDC7-ASK), JPO2 (also known as R1, RAM2 and CDCA7L) and pogo transposable element with zinc finger domain (PogZ) [30] , [31] , [32] , [33] . JPO2 is a 454-amino-acid protein that binds c-Myc via a leucine-zipper motif (amino-acid residues 213–235, Fig. 1 ) and contributes to c-Myc-mediated transformation in medulloblastoma [34] . It also acts as a transcriptional repressor of monoamino oxidases A and B by binding to promoter Sp1 elements [35] , [36] . PogZ is a domesticated transposase containing a predicted DDE domain at its C-terminus (residues 1,117–1,323; Fig. 1 ) [31] . This domain is typically present in enzymes that catalyse DNA cleavage followed by a strand transfer reaction. PogZ regulates the Aurora B kinase through interaction with heterochromatin protein 1, which is required for correct chromosome segregation during mitosis [37] . Like the HIV pre-integration and MLL1-menin complexes, JPO2 and PogZ are tethered to chromatin by LEDGF/p75 (refs 30 , 31 , 33 ). Despite intensive research focused on HIV IN and MLL1/menin interactions with the LEDGF/p75 IBD, the interaction mode of other physiological IBD-binding partners remained enigmatic. In this work, we characterized the interaction interfaces of both JPO2 and PogZ with the IBD revealing an overlap with the regions responsible for interactions with HIV IN and MLL1. Identification of a highly conserved consensus IBD-binding motif (IBM), present in all validated cellular IBD-interacting proteins, led to discovery of interacts-with-Spt6 (IWS1) as a novel binding partner. Moreover, our results show that the HIV IN interaction site on the IBD overlaps with that of PogZ, JPO2 and MLL1 but shows an alternative interaction mode explaining why HIV IN can efficiently outcompete endogenous interaction partners. JPO2 interacts with the IBD through a disordered region To characterize the interactions between the LEDGF/p75 IBD and JPO2, we expressed recombinant protein fragments in E. coli . A JPO2 construct encoding residues 1–130 (JPO2 1–130 ), including the specific LEDGF/p75 interaction domain described earlier (amino-acid residues 62–94 (ref. 33 ) or 77–98 (ref. 30 )), was most suitable for overexpression in E. coli ( Fig. 1 ). The IBD construct used in this study contains LEDGF/p75 residues 345–426. The C-terminal boundary was optimized based on analysis of the crystal structure of the IBD in complex with HIV-1 IN (PDB ID 2B4J [38] ). Inclusion of residues N425 and M426 at the C-terminus dramatically improved protein expression yields. Initially, we characterized the structural features of JPO2 1–130 in the absence of the IBD. Several lines of evidence led us to conclude that JPO2 1–130 is intrinsically disordered. In particular, circular dichroism (CD) spectra obtained for the fragment revealed the absence of regular secondary structure elements ( Fig. 2a ). In addition, evaluation of the protein’s thermal stability in various buffers using differential scanning fluorimetry (DSF) indicated the absence of a hydrophobic core ( Fig. 2b ). Interestingly, the fluorescence profile of the IBD-JPO2 1–130 complex suggested formation of a hydrophobic core ( Supplementary Fig. 1b ). Finally, 1D 1 H and two-dimensional (2D) 15 N/ 1 H HSQC NMR spectra of JPO2 1–130 showed poor dispersion of groups of signals that are usually well-dispersed in structured globular proteins ( Fig. 2c,d and Supplementary Fig. 2 ). Our experimental results indicating the lack of a regular JPO2 1–130 structure are in good agreement with bioinformatic analysis of JPO2 ( Supplementary Fig. 1e,f ). 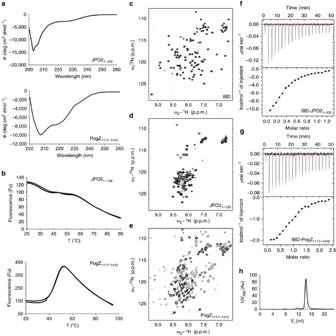Figure 2: Biophysical characterization of JPO21–130and PogZ1117–1410. (a) CD spectra of JPO21–130and PogZ1117–1410. (b) Fluorescence intensities of JPO21–130and PogZ1117–1410during DSF experiments. Two curves corresponding to experimental duplicates are shown. (c–e) Heteronuclear correlation NMR spectra obtained for the IBD (c), JPO21–130(d) and PogZ1117–1410(e). The unstructured character of JPO1–130(d) is clearly exhibited by the poor dispersion of its backbone amide signals compared with the well-dispersed signals of the structured constructs IBD (c) and the majority of PogZ1117–1410signals (e). (f,g) ITC data obtained for the IBD-JPO21–130and IBD-PogZ1117–1410interactions, respectively. Upper graph: experimental data; lower graph: fit (line) of the dilution-corrected integrated heats (full circles) from each injection of 60 μM JPO21–130or 114 μM PogZ1117–1410. (h) Analytical SEC analysis of PogZ1117–1410. Figure 2: Biophysical characterization of JPO2 1–130 and PogZ 1117–1410 . ( a ) CD spectra of JPO2 1–130 and PogZ 1117–1410 . ( b ) Fluorescence intensities of JPO2 1–130 and PogZ 1117–1410 during DSF experiments. Two curves corresponding to experimental duplicates are shown. ( c – e ) Heteronuclear correlation NMR spectra obtained for the IBD ( c ), JPO2 1–130 ( d ) and PogZ 1117–1410 ( e ). The unstructured character of JPO 1–130 ( d ) is clearly exhibited by the poor dispersion of its backbone amide signals compared with the well-dispersed signals of the structured constructs IBD ( c ) and the majority of PogZ 1117–1410 signals ( e ). ( f , g ) ITC data obtained for the IBD-JPO2 1–130 and IBD-PogZ 1117–1410 interactions, respectively. Upper graph: experimental data; lower graph: fit (line) of the dilution-corrected integrated heats (full circles) from each injection of 60 μM JPO2 1–130 or 114 μM PogZ 1117–1410 . ( h ) Analytical SEC analysis of PogZ 1117–1410 . Full size image The intrinsically disordered JPO2 1–130 fragment readily interacted with the IBD, forming a stable complex that could be isolated using size-exclusion chromatography (SEC; Supplementary Fig. 1g ). The low micromolar binding affinity ( K d =1.9±0.2 μM) of the complex was determined using isothermal titration calorimetry (ITC; Fig. 2f ). Interestingly, the stoichiometry of the interaction was estimated as two molecules of IBD per molecule of JPO2 1–130 (average N =1.9). PogZ dimers form a stable complex with the IBD The PogZ fragment used in this study (294 C-terminal residues; PogZ 1117–1410 ) includes the predicted DDE domain, which was previously identified as a region responsible for interaction with the IBD [31] ( Fig. 1 ). Domain boundaries were estimated based on secondary structure predictions and sequence homology between the DDE domain of PogZ and Mos1, a transposase with known crystal structure (PDB ID 2F7T [39] ). Biophysical characterization including 1 H NMR and 2D 15 N/ 1 H HSQC NMR spectra ( Fig. 2e and Supplementary Fig. 2 ) suggested that PogZ 1117–1410 adopts a well-defined conformation, although the presence of an unstructured region at the C-terminus (residues 1,373–1,410) was confirmed by limited proteolysis ( Supplementary Fig. 3a ) and by the presence of more than 30 backbone amide signals in the 2D 15 N/ 1 H HSQC spectrum that are considerably sharper and less well-dispersed than the majority of amide signals from the structured part of the protein. The structured character of PogZ 1117–1410 was further supported by CD spectra and DSF measurements. In particular, CD spectra revealed a substantial presence of α-helices and β-structures ( Fig. 2a ) and DSF showed a fluorescence profile typical for a folded protein with a hydrophobic core ( Fig. 2b ). In addition, PogZ 1117–1410 showed a significant increase in thermal stability in the presence of Mg 2+ , as evidenced by a titration experiment monitored by DSF ( Supplementary Fig. 3b ). This is in agreement with the known metal-binding properties of the predicted DDE domain in PogZ. To assess the affinity of PogZ 1117–1410 for the IBD, we used ITC ( Fig. 2g ). PogZ 1117–1410 binds the IBD with a K d of 1.6±0.2 μM and a 1:1 stoichiometry ( N =0.94). Analytical SEC indicated that PogZ 1117–1410 exists as a dimer in solution ( Fig. 2h ). The retention volume of PogZ 1117–1410 ( V r =14.24 ml) corresponded to a molecular weight of 64,600 Da according to the calibration trendline equation. This suggests dimeric assembly of PogZ 1117–1410 (theoretical molecular weight: 33,111 Da). Moreover, upon IBD binding the amide group signals from the structured regions of PogZ almost completely disappeared from the triple-resonance three-dimensional (3D) NMR spectra, as the 80 kDa assembly is over the detection limit of these experiments, while only signals from the relatively flexible C-termini can be observed in the spectra. Signals from these flexible regions are proportionally less affected by the molecular weight increase upon complex formation. Together, these data suggest that PogZ 1117–1410 forms a structured dimer with disordered C-termini. As analytical SEC indicated monomeric assembly of free IBD in solution ( Supplementary Fig. 3c ) and dimeric assembly of free PogZ 1117–1410 ( Fig. 2h ), each PogZ dimer forms a complex with two molecules of IBD. Interaction interfaces for cellular partners on IBD overlap We employed NMR spectroscopy for detailed characterization of the interactions of the IBD with JPO2 and PogZ. Overlays of the 2D 15 N/ 1 H HSQC spectra obtained for free 15 N-labelled IBD and 15 N-labelled IBD in complex with either JPO2 1–130 or PogZ 1117–1410 reveal significant shifts in the positions of backbone amide signals in both complexes ( Fig. 3a,b ). To interpret the changes in the IBD signal positions, we acquired essentially complete sequence-specific backbone resonance assignment of 13 C/ 15 N-labelled IBD using a set of standard triple-resonance NMR experiments. We assigned 95.4% of 1 H, 15 N, 13 C′ and 13 C α/β atoms of the IBD. Backbone amide signals ( 15 N and 1 H) were assigned for all residues except for four amino acids (E345, M348, Q410 and T417). There were no unassigned resolved spin systems detected in the spectra. 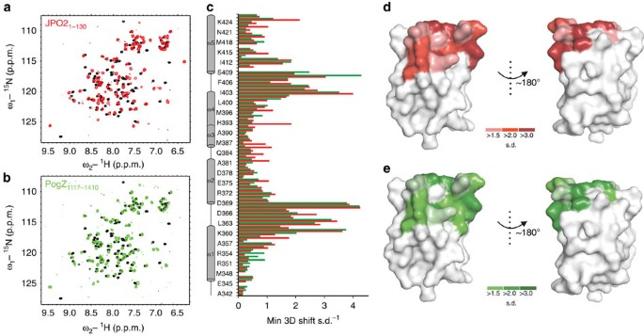Figure 3: Structural characterization of the interactions of the IBD with JPO21–130or PogZ1117–1410. Comparison of the 2D15N/1H HSQC spectra of free (black) and partner-bound IBD (red/green). The red spectrum in panel (a) was obtained from the complex of15N-labelled IBD with unlabelled JPO21–130; the green spectrum in panel (b) was obtained from the complex of15N-labelled IBD with unlabelled PogZ1117–1410. (c) IBD minimal chemical shift values divided by corresponding s.d. for backbone resonances (15N,13C′ and1HN) calculated for both complexes (red: IBD-JPO21–130; green IBD-PogZ1117–1410). α-helices of the IBD (α1–α5) are schematically illustrated. (d,e) Structural overview of specific changes induced in the positions of IBD backbone resonances by either JPO21–130(d) or PogZ1117–1410(e). Residues with substantial chemical shifts are highlighted on the IBD crystal structure (PDB ID 2B4J38). The colour saturation reflects the relative degree of chemical shift perturbations as a multiple of s.d. of the corresponding data set. Figure 3: Structural characterization of the interactions of the IBD with JPO2 1–130 or PogZ 1117–1410 . Comparison of the 2D 15 N/ 1 H HSQC spectra of free (black) and partner-bound IBD (red/green). The red spectrum in panel ( a ) was obtained from the complex of 15 N-labelled IBD with unlabelled JPO2 1–130 ; the green spectrum in panel ( b ) was obtained from the complex of 15 N-labelled IBD with unlabelled PogZ 1117–1410 . ( c ) IBD minimal chemical shift values divided by corresponding s.d. for backbone resonances ( 15 N, 13 C′ and 1 H N ) calculated for both complexes (red: IBD-JPO2 1–130 ; green IBD-PogZ 1117–1410 ). α-helices of the IBD (α1–α5) are schematically illustrated. ( d , e ) Structural overview of specific changes induced in the positions of IBD backbone resonances by either JPO2 1–130 ( d ) or PogZ 1117–1410 ( e ). Residues with substantial chemical shifts are highlighted on the IBD crystal structure (PDB ID 2B4J [38] ). The colour saturation reflects the relative degree of chemical shift perturbations as a multiple of s.d. of the corresponding data set. Full size image Formation of the IBD-JPO2 1–130 and IBD-PogZ 1117–1410 complexes was followed via chemical shift perturbations of IBD backbone signals ( 1 H, 15 N and 13 C′) induced by each binding partner in the 3D HNCO spectra. The specific changes induced by JPO2 1–130 and PogZ 1117–1410 overlapped significantly and were localized in two distinct regions in the IBD sequence ( Fig. 3c ). In particular, binding of JPO2 1–130 induced substantial changes in two regions of the IBD structure (residues I359–D369 and K402–M413) including two adjacent, surface-exposed interhelical loops ( Fig. 3d ). In addition, we identified a subset of residues within those two regions that showed the largest perturbations (N361, L363, K364, D366, L368, D369, I403, R404 and V408). These residues are most likely in direct contact with JPO2 1–130 ( Fig. 3d ). We found no evidence of structural changes induced by the binding of JPO2 1–130 in other parts of the IBD. Similarly, substantial changes in the positions of IBD backbone signals induced by PogZ 1117–1410 binding were localized in regions spanning residues K360–D369 and K402–I412. The residues most affected by PogZ 1117–1410 binding (N361, L363, K364, L368, D369, I403 and V408) were analogous to those contributing to JPO2 1–130 binding ( Fig. 3d ). Highly similar results were obtained previously for mapping of the IBD-MLL1 interaction [14] , indicating that JPO2, PogZ and MLL1 share a common interaction interface on IBD ( Supplementary Fig. 3d ). A linear consensus motif mediates the interaction with IBD Detailed mapping of the IBD-binding epitopes of JPO2 and PogZ was performed analogously to that of the IBD. Overlays of the 2D 15 N/ 1 H HSQC NMR spectra obtained for free 15 N-labelled JPO2 1–130 and PogZ 1117–1410 and those measured in complex with IBD revealed significant shifts in the backbone amide signal positions ( Fig. 4a,b ). Interestingly, the changes observed in the PogZ 1117–1410 spectrum were strictly limited to a subset of more intensive signals expected to represent the flexible unstructured C-terminal region of the protein. To gain further insight into the topology of these specific changes, we carried out sequence-specific backbone resonance assignment of 13 C/ 15 N-labelled JPO2 1–130 and PogZ 1117–1410 using a set of standard triple-resonance NMR experiments. We assigned 94.4% of 1 H, 15 N, 13 C′ and 13 C α/β atoms of JPO2 1–130 . For PogZ 1117–1410 , we were able to assign essentially all 1 H, 15 N, 13 C′ and 13 C α/β signals of an apparently unstructured C-terminal region (residues 1,368–1,410) that was significantly affected by IBD binding. 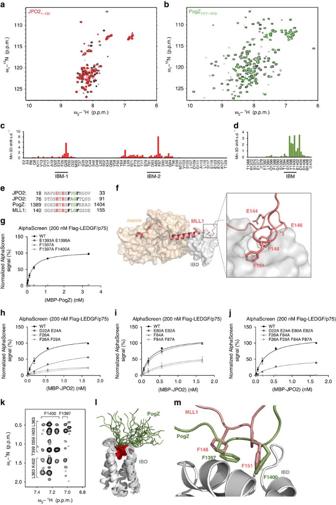Figure 4: The IBD-binding epitopes of PogZ and JPO2 are formed by a linear consensus motif. (a,b) Comparison of the 2D15N/1H HSQC spectra of the free (black) and IBD-bound (red)13C/15N-labelled JPO21–130(a) and PogZ1117–1410(b). (c,d) JPO21–130(c) and PogZ1117–1410(d) minimal chemical shift values divided by the corresponding s.d. for backbone resonances (15N,13C′ and1HN) calculated for the IBD-JPO21–130or IBD-PogZ1117–1410complexes. (e) Consensus IBM identified in LEDGF/p75 binding partners. (f) Model of the MLL1-menin-LEDGF/p75 ternary complex14. Menin is highlighted in orange, the LEDGF/p75 IBD in grey and MLL1 in pink. Amino-acid residues corresponding to the consensus motif (E144, E146, F148 and F151) are represented as sticks. (g) Mutations in the IBM of PogZ abolish the interaction with LEDGF/p75. Recombinant WT or mutant MBP-PogZ variants were titrated against Flag-LEDGF/p75 in AlphaScreen experiments. (h–j) AlphaScreens assessing LEDGF/p75 binding to JPO2 constructs with mutations in the first (h), second (i) or both IBMs (j). WT or mutant MBP-JPO2 variants were titrated against 200 nM Flag-LEDGF/p75. Error bars in all AlphaScreens represent s.d. calculated from three independent experiments, each performed in duplicate. (k) A region from the 2D13C/15N-filtered/edited NOESY spectrum obtained for the IBD-PogZ1389–1404complex. The spectrum shows intermolecular NOE contacts between13C/15N-labelled IBD and unlabelled PogZ1389–1404. (l) Converged structures of IBD-PogZ1389–1404complex as determined by NMR (PDB ID: 2n3a). F1397 and F1400 are depicted as red sticks. (m) Detailed view of the IBD-PogZ1389–1404binding interface (PDB ID: 2n3a) in comparison with the one of MLL140–160(PDB ID: 2msr14). Representative NMR structures are shown. Figure 4: The IBD-binding epitopes of PogZ and JPO2 are formed by a linear consensus motif. ( a , b ) Comparison of the 2D 15 N/ 1 H HSQC spectra of the free (black) and IBD-bound (red) 13 C/ 15 N-labelled JPO2 1–130 ( a ) and PogZ 1117–1410 ( b ). ( c , d ) JPO2 1–130 ( c ) and PogZ 1117–1410 ( d ) minimal chemical shift values divided by the corresponding s.d. for backbone resonances ( 15 N, 13 C′ and 1 H N ) calculated for the IBD-JPO2 1–130 or IBD-PogZ 1117–1410 complexes. ( e ) Consensus IBM identified in LEDGF/p75 binding partners. ( f ) Model of the MLL1-menin-LEDGF/p75 ternary complex [14] . Menin is highlighted in orange, the LEDGF/p75 IBD in grey and MLL1 in pink. Amino-acid residues corresponding to the consensus motif (E144, E146, F148 and F151) are represented as sticks. ( g ) Mutations in the IBM of PogZ abolish the interaction with LEDGF/p75. Recombinant WT or mutant MBP-PogZ variants were titrated against Flag-LEDGF/p75 in AlphaScreen experiments. ( h – j ) AlphaScreens assessing LEDGF/p75 binding to JPO2 constructs with mutations in the first ( h ), second ( i ) or both IBMs ( j ). WT or mutant MBP-JPO2 variants were titrated against 200 nM Flag-LEDGF/p75. Error bars in all AlphaScreens represent s.d. calculated from three independent experiments, each performed in duplicate. ( k ) A region from the 2D 13 C/ 15 N-filtered/edited NOESY spectrum obtained for the IBD-PogZ 1389–1404 complex. The spectrum shows intermolecular NOE contacts between 13 C/ 15 N-labelled IBD and unlabelled PogZ 1389–1404 . ( l ) Converged structures of IBD-PogZ 1389–1404 complex as determined by NMR (PDB ID: 2n3a). F1397 and F1400 are depicted as red sticks. ( m ) Detailed view of the IBD-PogZ 1389–1404 binding interface (PDB ID: 2n3a) in comparison with the one of MLL 140–160 (PDB ID: 2msr [14] ). Representative NMR structures are shown. Full size image The effects of complex formation on individual amino-acid residues of JPO2 1–130 and PogZ 1117–1410 were quantified as minimal chemical shift values in backbone resonances ( 15 N, 13 C′ and 1 H N ) divided by corresponding s.d. ( Fig. 4c,d ). In the highly overlapping spectra of the unstructured JPO2 1–130 , we were able to discern seven significantly affected residues (V27, G28, F29, T66, G86, F87 and N93). In the case of PogZ 1117–1410 , the most affected residues (F1397, Y1398, G1399, F1400 and A1403) were recognized in a single stretch at the C-terminus. Alignment of the sequences encompassing these residues with the recently published IBD-interacting residues of MLL1 (residues 140–155) [14] revealed a conserved consensus sequence ((E/D)-X-E-X-F-X-G-F), which we refer to as the IBM ( Fig. 4e ). Interestingly, JPO2 contains two of these motifs, IBM-1 (D22-F29) and IBM-2 (E80-F87), while both MLL1 (E144-F151) and PogZ (E1393-F1400) contain only one. Two phenylalanine residues in the IBM of MLL1 have been shown to play a key role in binding to LEDGF/p75; residues F148 and F151 anchor a MLL1-derived peptide in two hydrophobic pockets on the IBD surface in a model of the MLL1/menin-IBD complex ( Fig. 4f ), and their mutation abrogates the interaction with LEDGF/p75 (ref. 14 ). We introduced a F1397A point mutation (PogZ F1397A ) or a double F1397A/F1400A mutation (PogZ F1397A/F1400A ) into recombinant maltose binding protein (MBP)-tagged PogZ 1117–1410 and evaluated the interactions of these mutants with Flag-tagged LEDGF/p75 in an AlphaScreen assay ( Fig. 4g ). These mutations abolished the interaction of the PogZ fragment with LEDGF/p75. Corresponding single and double mutations were introduced in both IBMs of MBP-tagged JPO2 (IBM-1: JPO2 F26A and JPO2 F26A/F29A ; IBM-2: JPO2 F84A and JPO2 F84A/F87A ) and analysed for their interactions with Flag-LEDGF/p75 ( Fig. 4h,i ). Although these mutations affected the interaction with Flag-LEDGF/p75, they were not sufficient to fully disrupt it. This suggests that both IBM-1 and IBM-2 contribute to the interaction of JPO2 with LEDGF/p75. Mutations of phenylalanines in both motifs (JPO2 F26A/F84A or JPO2 F26A/F29A/F84A/F87A ) fully abolished the interaction of JPO2 with LEDGF/p75 ( Fig. 4j ). The fact that mutation of phenylalanine residues in the IBM is sufficient to abrogate the interaction is in agreement with previous data obtained for MLL1 (ref. 14 ). The glycine at position seven in the IBM is most likely conserved owing to its ability to reduce steric hindrance. However, the reason for conservation of the glutamic/aspartic acid residues in positions one and three is less clear. An interaction between this part of the consensus motif and the IBD was not detected in the NMR experiments with JPO2, PogZ ( Fig. 4 ) or MLL1 (ref. 14 ). To assess the importance of these residues in LEDGF/p75 interactions, we mutated them to alanines. While PogZ E1393A/E1395A did not interact with LEDGF/p75 ( Fig. 4g ), single IBM mutations in JPO2 (JPO2 D22A/E24A or JPO2 E80A/E82A ) disrupted the interaction only partially ( Fig. 4h,i ). Combining mutations in both IBMs of JPO2 (JPO2 D22A/E24A/E80A/E82A ) reduced the interaction further, supporting the notion that both JPO2 IBMs can bind LEDGF/p75 ( Fig. 4j ). The introduced mutations and their effects on LEDGF/p75 binding are summarized in Supplementary Table 1 . Taken together, these results establish the existence of an unstructured conserved protein motif responsible for interaction with the LEDGF/p75 IBD. Structural validation of the consensus motif To provide a more detailed insight into the actual organization of the interaction interface, initially mapped by backbone NMR signal perturbations, we solved the solution structure of the PogZ-derived peptide in complex with the IBD (PDB ID: 2n3a), as a representative of the IBM. In particular, we determined the solution structure of the PogZ-derived peptide (PogZ 1389–1404 ) in complex with the IBD using the previously published approach [14] . Comprehensive backbone and side-chain resonance assignments for the PogZ 1389–1404 bound 13 C/ 15 N labelled LEDGF/p75 IBD were obtained using established triple-resonance experiments and for the bound unlabelled PogZ 1389–1404 peptide using 13 C/ 15 N filtered homonuclear total correlation spectroscopy and nuclear Overhauser enhancement spectroscopy (NOESY) experiments. The essentially complete 15 N, 13 C and 1 H resonance assignments allowed automated assignment of the nuclear Overhauser effects (NOEs) identified in 3D 15 N/ 1 H NOESY-HSQC, 13 C/ 1 H HSQC-NOESY and in 2D 13 C/ 15 N-filtered/edited NOESY spectra using the protocol implemented in Cyana. This yielded unique assignments for 94.9% (1878/1978) of the NOE peaks observed, providing 1,018 non-redundant 1 H– 1 H distance constraints, including 35 intermolecular constraints ( Fig. 4k ). Forty converged structures for the IBD-PogZ 1389–1404 complex with no distance violations >0.2 Å were obtained from 100 random starting conformations using 1,156 NMR-derived structural constraints ( ∼ 13.6 constraints per restrained residue). The 29 lowest energy conformers were further refined in explicit solvent in YASARA ( Fig. 4l ). Structural statistics for the final water-refined set of structures are shown in Supplementary Table 2 . Analogously to our recently published work on the MLL-LEDGF/p75 interaction [14] , detailed analysis of the NOESY data revealed that the interaction of PogZ 1389–1404 with the IBD is maintained mainly by the aromatic side chains of two phenylalanine residues (F1397 and F1400) within the linear IBM ( Fig. 4m ). As expected, the IBD adopts a well-defined conformation, while PogZ 1389–1404 remains relatively unstructured. PogZ 1389–1404 is anchored between the two interhelical loops of IBD (aa I359 to D369 and K402 to M413) via F1397 and F1400 in a similar manner as MLL1 140–160 , as illustrated by a comparison of the structural data obtained for both complexes shown in Fig. 4m . IWS1 is a novel interacting partner of LEDGF/p75 Next, we used the ScanProsite [40] algorithm to identify additional proteins containing the IBM sequence. In addition to MLL1, JPO2 and PogZ, we found the motif in the known LEDGF/p75 interaction partners MLL2 (ref. 41 ) and ASK (DBF4) from the CDC7-ASK complex [32] . Moreover, IBM and IBM-like motifs were found in the mediator complex subunit 1 (Med1; residues 891–898) and IWS1 (residues 484–491; Fig. 5a,b ). Three other IBM-containing proteins: eukaryotic translation initiation factor 4H (eiF4H), ATP-binding cassette transporter 1 (ABCA1) and retinitis pigmentosa 1 protein (RP1) were excluded from further studies based on their structures, extranuclear localization and physiological roles. 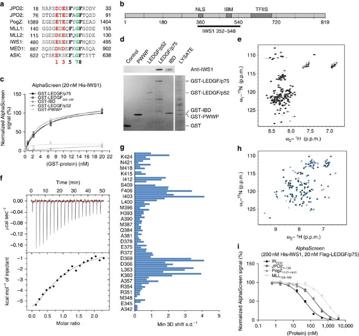Figure 5: LEDGF/p75 interacts with IWS1. (a) Alignment of the IBM and IBM-like motifs identified in human nuclear proteins. Conserved positions are numbered. (b) Domain organization of IWS1. The IWS1352–548fragment is highlighted by a black bar below the scheme. The transcription elongation factor S-II domain, the nuclear localization signal5and the IBM are indicated. (c) IWS1 interacts exclusively with LEDGF/p75 constructs containing the IBD. Recombinant GST-LEDGF/p75, GST-LEDGF/p75325–530, GST-IBD, GST-PWWP or GST-LEDGF/p52 were titrated against 20 nM His-IWS1 in AlphaScreen. Error bars represent s.d. calculated from three independent experiments, each performed in duplicate. (d) Pull down of endogenous IWS1 from SupT1 nuclear lysate using GST (control), GST-PWWP, GST-LEDGF/p52, GST-LEDGF/p75 or GST-IBD as bait. The nuclear lysate and LEDGF/p75 fragments were analysed by Coomassie staining. IWS1 was detected by western blot using anti-IWS1 antibody. (e) 2D15N/1H HSQC NMR spectra obtained for IWS1352–548.The unstructured character of IWS1352–548is illustrated by the poor dispersion of amide signals. (f) ITC data obtained for the IBD-IWS1352–548interaction. Upper graph: experimental data; lower graph: fit of the dilution-corrected integrated heat data (full circles) from each injection of 145 μM IWS1352–548. (g,h) Characterization of the IBD-IWS1352–548interaction. (g) Comparison of the 2D15N/1H HSQC spectra of the free (black) and IWS1352–548-bound (blue)15N-labelled IBD. (h) Minimal chemical shift values divided by the corresponding s.d. for IBD backbone resonances (15N,13C′ and1HN) calculated for the IBD-IWS1352–548complex. (i) HIV-1 INCCD, JPO21–130, PogZ1117–1410and MLL1123–160protein fragments interfere with LEDGF/p75-IWS1 complex formationin vitro. The interaction between recombinant full-length Flag-LEDGF/p75 (20 nM) and His-IWS1 (200 nM) was monitored in an AlphaScreen assay, while an increasing amount of untagged INCCD, JPO21–130, PogZ1117–1410or MLL1123–160protein fragments were added. Error bars represent s.d. calculated from two independent experiments performed in duplicate. Figure 5: LEDGF/p75 interacts with IWS1. ( a ) Alignment of the IBM and IBM-like motifs identified in human nuclear proteins. Conserved positions are numbered. ( b ) Domain organization of IWS1. The IWS1 352–548 fragment is highlighted by a black bar below the scheme. The transcription elongation factor S-II domain, the nuclear localization signal [5] and the IBM are indicated. ( c ) IWS1 interacts exclusively with LEDGF/p75 constructs containing the IBD. Recombinant GST-LEDGF/p75, GST-LEDGF/p75 325–530 , GST-IBD, GST-PWWP or GST-LEDGF/p52 were titrated against 20 nM His-IWS1 in AlphaScreen. Error bars represent s.d. calculated from three independent experiments, each performed in duplicate. ( d ) Pull down of endogenous IWS1 from SupT1 nuclear lysate using GST (control), GST-PWWP, GST-LEDGF/p52, GST-LEDGF/p75 or GST-IBD as bait. The nuclear lysate and LEDGF/p75 fragments were analysed by Coomassie staining. IWS1 was detected by western blot using anti-IWS1 antibody. ( e ) 2D 15 N/ 1 H HSQC NMR spectra obtained for IWS1 352–548. The unstructured character of IWS1 352–548 is illustrated by the poor dispersion of amide signals. ( f ) ITC data obtained for the IBD-IWS1 352–548 interaction. Upper graph: experimental data; lower graph: fit of the dilution-corrected integrated heat data (full circles) from each injection of 145 μM IWS1 352–548 . ( g , h ) Characterization of the IBD-IWS1 352–548 interaction. ( g ) Comparison of the 2D 15 N/ 1 H HSQC spectra of the free (black) and IWS1 352–548 -bound (blue) 15 N-labelled IBD. ( h ) Minimal chemical shift values divided by the corresponding s.d. for IBD backbone resonances ( 15 N, 13 C′ and 1 H N ) calculated for the IBD-IWS1 352–548 complex. ( i ) HIV-1 IN CCD , JPO2 1–130 , PogZ 1117–1410 and MLL1 123–160 protein fragments interfere with LEDGF/p75-IWS1 complex formation in vitro . The interaction between recombinant full-length Flag-LEDGF/p75 (20 nM) and His-IWS1 (200 nM) was monitored in an AlphaScreen assay, while an increasing amount of untagged IN CCD , JPO2 1–130 , PogZ 1117–1410 or MLL1 123–160 protein fragments were added. Error bars represent s.d. calculated from two independent experiments performed in duplicate. Full size image IWS1 forms a complex with transcription elongation factor SPT6 and the C-terminal domain (CTD) of the large subunit of RNA polymerase II (RNAPII). This complex recruits HYPB/Setd2 histone methyltransferase, which controls H3K36me3 methylation, affecting co-transcriptional pre-mRNA splicing and export [42] , [43] . Because LEDGF is linked to both alternative splicing and interaction with H3K36me3, we chose to experimentally investigate the interaction between LEDGF/p75 and IWS1. We evaluated the binding of recombinant His-tagged full-length IWS1 (His-IWS1) to various GST-tagged LEDGF deletion mutants using AlphaScreen. His-IWS1 interacted exclusively with LEDGF/p75 fragments containing the IBD (full-length GST-LEDGF/p75, GST-LEDGF/p75 325–530 and GST-IBD; ( Figs 1 and 5c ). The interaction between IWS1 and LEDGF/p75 was corroborated by results from a pull-down experiment. GST-tagged LEDGF/p75, LEDGF/p52, PWWP or IBD were immobilized on glutathione sepharose resin and incubated with nuclear extracts of SupT1 cells. IWS1 could only be pulled down by GST-LEDGF/p75 and GST-IBD ( Fig. 5d ). To obtain additional insight into the IWS1-LEDGF/p75 interaction, we cloned, expressed and purified a fragment of IWS1 containing the predicted IBM and encoding residues 352–548 (IWS1 352–548 ; Fig. 5b ). Fragment boundaries were based on computational analyses including domain and repeat profiling and secondary structure, disorder and hydrophobicity predictions. These predictions indicated that IWS1 residues 1–550 are unstructured and contain a highly acidic Glu-rich region (residues 83–509; Supplementary Fig. 4a,b ). The unstructured character of the fragment was verified experimentally using CD spectroscopy, DSF and 1D 1 H and 2D 15 N/ 1 H HSQC NMR spectra ( Fig. 5e , Supplementary Figs 2 and 4c,d ). Under optimal conditions (25 mM Tris-HCl, pH 8.5, 150 mM NaCl, 0.05% BME), the IBD-IWS1 352–548 complex could readily be isolated using analytical SEC ( Supplementary Fig. 4d ), and the affinity of the interaction was determined using ITC ( Fig. 5f ). We calculated a K d value of 6.7±2.0 μM and a 1:1 binding stoichiometry ( N =0.96). We followed the formation of the IBD-IWS1 352–548 complexes via chemical shift perturbations of the IBD backbone signals ( 1 H, 15 N, 13 C′; Fig. 5g ) in the 3D HNCO spectra, analogous to our experiments with JPO2 1–130 and PogZ 1117–1410 . The specific changes induced by IWS1 352–548 were localized to residues K360–D369, K402–V408, I412 and M413 of the IBD and overlap with those found for JPO2, PogZ and MLL1 ( Fig. 5h ). Overall, these experiments unambiguously confirm a novel IBM-mediated interaction between IWS1 and the LEDGF/p75 IBD. As published earlier, the binding of HIV-1 integrase, JPO2, PogZ and MLL1 to LEDGF/p75 is mutually exclusive [14] , [30] , [31] . Our NMR data confirmed that IWS1 also shares the same interface on the IBD ( Fig. 5g,h ). Therefore, we evaluated the effect of HIV-1 integrase catalytic core domain (IN CCD ), JPO2 1–130 , PogZ 1117–1410 and MLL1 123–160 titration on the LEDGF/p75-IWS1 interaction in an AlphaScreen assay. As shown in Fig. 5i , untagged IN CCD , JPO2 1–130 , PogZ 1117–1410 and MLL1 123–160 efficiently displaced IWS1 from the LEDGF/p75-IWS1 complex. Apparent 50% inhibitory concentrations (IC 50 ) were: 46 nM for IN CCD (95% confidence interval (CI) (36; 59)), 184 nM for JPO2 1–130 (95% CI (153; 221)), 209 nM for PogZ 1117–1410 (95% CI (162; 269)) and 848 nM for MLL1 123–160 (95% CI (612; 1,175)). As described above, we obtained dissociation constants for the three studied LEDGF/p75 binding partners (JPO2 1–130 1.6 μM, PogZ 1117–1410 1.9 μM and IWS1 352–548 6.7 μM) using ITC. The K d of LEDGF—IN and MLL1—LEDGF interactions were reported earlier and are 10.9 nM and 86.3 μM, respectively [14] , [44] . The K d and IC 50 values follow the same trend with IN CCD having higher affinity than the physiological binding partners. HIV IN, JPO2 and PogZ are known to co-localize with LEDGF/p75 on the chromatin of the cell [16] , [30] , [31] , [33] . To investigate potential LEDGF/p75-IWS1 co-localization, HeLa cells were transfected with a Flag-tagged IWS1 (Flag-IWS1) expression construct and stained for endogenous LEDGF/p75 and the Flag-tag ( Supplementary Fig. 5a ). As shown before LEDGF/p75 displayed a dense fine speckled distribution in interphase cells and remained attached to chromatin during mitosis. Flag-tagged IWS1 also localized to the nucleus of the cell but showed a more equal distribution compared with endogenous LEDGF/p75 ( Supplementary Fig. 5a ). Flag-IWS1 did not co-localize extensively with LEDGF/p75 in the interphase and did not bind mitotic chromatin. However, under the same conditions Flag-tagged HIV IN and JPO2 did co-localize extensively with LEDGF/p75 ( Supplementary Fig. 6a ) consistently with previously published results [16] , [30] , [31] , [33] . Neither overexpression of eGFP-LEDGF/p75 ( Supplementary Fig. 7 ), or stable knockdown of LEDGF/p75 (95% as determined by Q-RT-PCR; Supplementary Fig. 5a ) did alter the cellular distribution of Flag-IWS1. This is in contrast to earlier reports on the LEDGF/p75 interactors JPO2 and HIV IN [30] , [33] , [45] . During the reviewing process of this manuscript Gérard et al ., reported on the interaction between LEDGF/p75 and IWS1 and revealed its role in HIV latency [46] . IWS1 is known to form a stable complex with the Suppressor of Ty6 (Spt6) and Gerard et al . could confirm the presence of a LEDGF/p75-IWS1-Spt6 triple complex. We confirmed a direct interaction between recombinant His-tagged IWS1 (His-IWS1) and a GST-tagged Spt6 fragment (GST-Spt6 194–230 ) in the absence of LEDGF/p75 in an AlphaScreen assay ( Supplementary Fig. 5b ) [47] . In addition, we could observe extensive co-localization between HA-tagged IWS1 and Flag-Spt6 ( Supplementary Fig. 6b ). Direct interaction between LEDGF/p75 and SPT6 could not be detected by AlphaScreen or pull-down experiments. However, these experiments confirmed the existence of the LEDGF/p75-IWS1-Spt6 ternary complex ( Supplementary Fig. 5c,d ). Co-expression of Spt6 did not increase the co-localization of Flag-IWS1 with eGFP-LEDGF/p75 in HeLa cells ( Supplementary Fig. 6c ). The IBD-IBM interaction is mimicked by lentiviral integrases Our structural analysis revealed that MLL1, JPO2 and PogZ interact with the same binding site on the IBD through their IBMs. This binding site is formed mainly by residues from two adjacent interhelical loops connecting IBD helices α1-α2 and α4-α5. The actual binding site consists of a basic surface created by positively charged residues (R404, R405, K407; Fig. 6a ) and two hydrophobic pockets (I359, K360, L363, L368, T399, K402, I403, F406, K407 and V408). These hydrophobic pockets are occupied by the conserved IBM phenylalanines, represented by MLL1 F148 and F151 ( Fig. 6b ). Electrostatic complementarity between the basic patch on the IBD and acidic residues of the IBM, represented by E144 and E146 of MLL1, further contributes to binding ( Fig. 6a ). 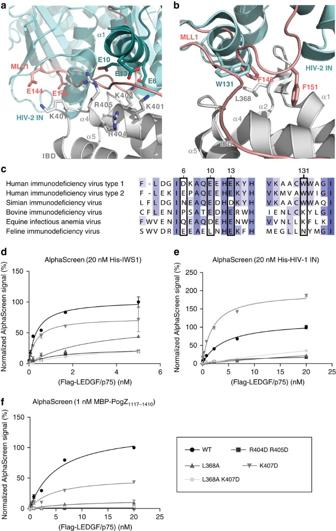Figure 6: Lentiviral integrases and LEDGF/p75 cellular binding partners recognize LEDGF/p75 via similar molecular mechanism. (a,b) Comparison of the bipartite interfaces of the MLL1-IBD and HIV-2 IN-IBD complexes (PDB IDs: 2MSR14, 3F9K48, respectively). The basic patch on the IBD recognized by HIV-2 IN E10 and MLL1 E144 (a) and the hydrophobic pocket recognized by HIV-2 IN W131 and MLL1 F148 (b). (c) Partial amino-acid sequence alignment of lentiviral integrases including residues of NTD and CCD responsible for interaction with LEDGF/p75 IBD. Conserved residues are coloured according to percentage of identity. Amino-acid residues corresponding to HIV-2 IN E6, E10, E13 and W131 are boxed. (d–f) Interaction of IWS1, JPO2, PogZ1117–1410or HIV-1 IN with LEDGF/p75 mutants defective for binding to MLL1 (R404D/R405D, L368A, K407D or L368A/K407D14). The interactions between recombinant WT His-IWS1 (d), His-HIV IN (e), MBP-PogZ1117–1410(f) and WT or mutant Flag-LEDGF/p75 were analysed by AlphaScreen. Error bars represent s.d. calculated from three independent experiments, each performed in duplicate. Figure 6: Lentiviral integrases and LEDGF/p75 cellular binding partners recognize LEDGF/p75 via similar molecular mechanism. ( a , b ) Comparison of the bipartite interfaces of the MLL1-IBD and HIV-2 IN-IBD complexes (PDB IDs: 2MSR [14] , 3F9K [48] , respectively). The basic patch on the IBD recognized by HIV-2 IN E10 and MLL1 E144 ( a ) and the hydrophobic pocket recognized by HIV-2 IN W131 and MLL1 F148 ( b ). ( c ) Partial amino-acid sequence alignment of lentiviral integrases including residues of NTD and CCD responsible for interaction with LEDGF/p75 IBD. Conserved residues are coloured according to percentage of identity. Amino-acid residues corresponding to HIV-2 IN E6, E10, E13 and W131 are boxed. ( d – f ) Interaction of IWS1, JPO2, PogZ 1117–1410 or HIV-1 IN with LEDGF/p75 mutants defective for binding to MLL1 (R404D/R405D, L368A, K407D or L368A/K407D [14] ). The interactions between recombinant WT His-IWS1 ( d ), His-HIV IN ( e ), MBP-PogZ 1117–1410 ( f ) and WT or mutant Flag-LEDGF/p75 were analysed by AlphaScreen. Error bars represent s.d. calculated from three independent experiments, each performed in duplicate. Full size image Structural comparison of the complexes of the IBD with the IBM of MLL1 (ref. 14 ) or HIV-2 IN [48] shows considerable overlap of both parts of the interface ( Fig. 6a,b ). One of the hydrophobic pockets on the IBD surface is occupied by W131 from the HIV-2 IN CCD ( Fig. 6b ). The basic surface of LEDGF/75 is recognized by the IN N-terminal domain (NTD). Specifically, acidic residues E6, E10, and E13 from the α1 helix of the HIV-2 IN NTD face positively charged residues K401, K402, R404 and R405 on the IBD α4 helix ( Fig. 6b ). The IN NTD-LEDGF/p75 interface is necessary for lentiviral integration [48] . In particular, LEDGF/p75 residues K401, R404 and R405 have a crucial role in HIV infectivity [48] . Their counterparts, corresponding to E10 and E13 of HIV-2 IN, are conserved among all lentiviral integrases ( Fig. 6c ). To further confirm the overlap of the IBD-binding interfaces of HIV-1 IN and other LEDGF/p75 interaction partners, we tested the binding of LEDGF/p75 mutants defective for interaction with MLL1 (ref. 14 ) to IWS1, PogZ 1117–1410 or HIV-1 IN. These mutations included L368A, which was expected to disrupt the hydrophobic interactions with the IBM phenylalanines or HIV IN tryptophan. R404D, R405D and K407D mutations were designed to target the electrostatic interactions. As expected, the L368A LEDGF/p75 mutant displayed reduced interactions with all binding partners ( Fig. 6 ). A similar effect was seen for LEDGF/p75 containing the R404D/R405D double mutation, which is known to affect interaction with HIV-2 IN E10 ( Fig. 6 ). These results underline the importance of these residues for LEDGF/p75 binding to many interaction partners and confirm features of the overlapping interface. On the other hand, LEDGF/p75 K407 contacts negatively charged side chains of MLL1 but does not establish contact with HIV IN [14] . Indeed, introduction of a K407D mutation negatively affected the interaction of LEDGF/p75 with IWS1 and PogZ 1117–1410 but increased its binding to HIV-1 IN ( Fig. 6 ). In addition, the K407D mutation slightly increased the effect of the L386A mutation on His-IWS1 and MBP-PogZ 1117–1410 binding ( Fig. 6 ). The PogZ and IWS1 IBMs thus exhibit similar properties as the MLL1 IBM in binding to LEDGF/p75 L368A and K407D [14] . In conclusion, although the binding mode of HIV IN to the IBD is not identical to that of the cellular binding partners, it uses the same basic surface and one of the hydrophobic pockets. LEDGF/p75 is a highly conserved protein present in all vertebrates. In addition, a protein harbouring PWWP and IBD-like domains can be found in arthropods and nematodes such as Drosophila melanogaster and Caenorhabditis elegans [49] . This conservation, together with the perinatal mortality observed in Psip1 knockout mice proves a crucial physiological role for LEDGF/p75 (ref. 3 ). LEDGF/p75 is tethered to chromatin through its AT-hooks and the PWWP domain, which recognizes H3K36me3 histone marks ( Fig. 1 ) [1] , [50] , [51] . Although LEDGF/p75-dependent chromatin tethering is essential for MLL1 fusion-driven leukaemia and HIV integration, a direct link to H3K36me3 marks has not yet been established. Likewise, the link between H3K36me3 marks and the potential cellular roles of LEDGF/p75 in DNA damage repair and pre-mRNA processing is not clear. Along with the PWWP domain, the IBD has a key role in the known physiological and pathological functions of LEDGF/p75 by mediating its interactions with various cellular and viral proteins [30] , [31] , [32] , [52] . Before this work, the interactions of a diverse set of proteins with the IBD were not fully understood, despite their importance to the development of therapies targeting LEDGF/p75 interactions to block MLL fusion-mediated leukaemic transformation and HIV integration [53] , [54] . Our results revealed that JPO2 and PogZ interact with the IBD through an intrinsically unstructured motif also found in MLL1 (ref. 14 ). Fragments of JPO2 and PogZ formed stable complexes with the IBD with affinities in the low micromolar range (1.6–1.9 μM) as measured by ITC. NMR experiments revealed that the IBD interaction interfaces for JPO2 1–130 and PogZ 1117–1410 are almost identical to the menin-independent MLL1 interface [14] . These interactions are maintained by two phenylalanine side chains occupying two hydrophobic pockets on the IBD. The first pocket is formed by IBD residues L363, L368, I403, F406, K407 and V408, while the second is formed by I359, K360, L363, T399, K402 and I403. Sequence alignment of the IBD-interacting regions of JPO2, PogZ and MLL1 revealed a consensus IBM ((E/D)-X-E-X-F-X-G-F), which was validated through comprehensive mutational analysis. IBMs were also identified in two other established LEDGF/p75 binding partners (MLL2 and CDC7-ASK) [32] , [52] . The consensus motif harbours two phenylalanine residues; the second phenylalanine is preceded by a glycine, most likely to avoid steric hindrance. These features of the IBM and its binding to IBD were validated by structural analysis of a novel IBD-PogZ 1389–1404 complex solution structure. Direct comparison of the IBD-PogZ 1389–1404 complex with the structure obtained for the MLL1-derived peptide containing the IBM (PDB ID: 2msr [14] ) therefore validates the conservation of the interactions mediated by the IBM ( Fig. 4m ). Several glutamic and aspartic acid residues precede the F-X-G-F segment of the motif. Although the interaction of these residues with IBD was not directly detected in any of the PogZ, JPO2 or MLL1 NMR experiments, mutagenesis experiments showed their complex-stabilizing effect in AlphaScreen assays. Interestingly, the CDC7-ASK IBM does not have a glutamic or aspartic acid residue at position 3, but it contains a glutamic acid at position 4 ( Fig. 5a ). In PogZ, the consensus motif was identified near the C-terminus, spanning residues E1393-F1400 ( Fig. 5a ). Mutational analysis confirmed that the phenylalanine residues are essential to maintain the interaction with LEDGF/p75. Likewise, mutation of both conserved glutamic acid residues to alanines abrogated the interaction. While PogZ-like proteins can be found in all bilateria, the IBM is apparently only present in bony vertebrates ( Supplementary Fig. 8 ). Surprisingly, JPO2 contains two IBMs encoded by the second and third exon ( Fig. 5a ). The presence of two IBMs is in agreement with results from our NMR and ITC experiments, which show an IBD: JPO2 1–130 stoichiometry of 2:1. Mutational analysis revealed that both motifs can interact with full-length LEDGF/p75 and that phenylalanines from both IBMs had to be mutated to abrogate the interaction. In contrast to PogZ, simultaneous mutation of D22, E24, E80 and E82 to alanines was not sufficient to fully abrogate the interaction. As the IBM of PogZ does not contain neighbouring glutamic and aspartic acid residues, E1394 and E1396 mutations have a more dramatic effect on LEDGF/p75 binding. Like LEDGF/p75 and PogZ, JPO2 is also evolutionally conserved among chordates. The presence of both JPO2 IBM motifs, however, seems to be more variable. While most species contain two motifs, Xenopus tropicalis and Gallus gallus have lost both motifs ( Supplementary Fig. 8 ). In each case, the absence of one or both copies of the motif coincides with a loss of the N-terminal portion of JPO2. Overall, the IBMs of LEDGF/p75 cellular interaction partners are conserved among chordates, suggesting important physiological roles for these interactions. IBM represents a typical example of Short linear motif (SLiM), a conserved amino-acid sequence present in natively disordered parts of the proteins that mediate binding independently of a larger sequence [55] . SLiMs are responsible for transient protein–protein interactions and owing to their limited intramolecular contacts with their partners, they tend to bind with low affinity. The short length and the disordered character of these regions provide a high level of plasticity, which makes SLiMs suitable elements to tune the functions of various eukaryotic regulatory proteins. On the other hand, such features also allow SLiMs to be imitated by pathogenic organisms. The ability to mimic the physiological interactions carried out via SLiMs is one of the ways employed by pathogens to take advantage of host cell functions and to guarantee their replication [56] . HIV-1 integrase is one of numerous viral proteins that evolved the ability to bind a cellular protein in a similar way as its cellular binding partners and exploit its physiological function. PogZ 1117–1410 forms dimers in solution as documented by analytical SEC, similar to Mos-1 DNA transposase the closest enzymatically active structural homologue of PogZ [31] . Together with our ITC stoichiometry results, this suggests the presence of two LEDGF/p75 molecules in the complex. Owing to the presence of two IBMs in JPO2, the JPO2-LEDGF/p75 complex presumably also contains two LEDGF/p75 molecules. A stable tetramer of HIV IN also has been shown to associate with two molecules of LEDGF/p75 (ref. 16 ). As such, it is tempting to speculate that multiple LEDGF/p75 molecules are needed to form a functional complex. A recent study reporting LEDGF/p75 dimers bound to certain DNA topologies [57] supports this hypothesis. In contrast, IWS1, MLL1 and CDC7-ASK dimers have not been described to date. However, some MLL1 fusions induce dimerization of the fusion protein. For these particular fusions, dimerization is required to maintain the transformed state [58] . In addition to the known LEDGF/p75 cellular interaction partners, several other human proteins contain IBMs (IWS1, Med1, eiF4H, ABCA1 and RP1). While the IBMs of Med1 and IWS1 are unstructured, as determined by structural predictions and NMR, respectively, the IBMs of other proteins are situated in predicted structured regions. As all the IBMs known so far are located in unstructured regions, we focused on the IWS1 protein. Intrinsically disordered proteins lack 3D structure yet carry out specific biological functions [59] . Typical intrinsically disordered proteins provide a platform for transient complex interactions between signalling and regulatory proteins. In eukaryotes, these interactions are especially important in transcription and its regulation [59] , [60] . IWS1 forms a stable complex with SPT6 and the CTD of the large subunit of RNAPII [42] . In addition, IWS1 has been shown to recruit HYPB/Setd2, the only histone methyltransferase known to create H3K36me3 marks [43] . The unstructured character of IWS1 was experimentally verified via comprehensive biophysical characterization. Next, we confirmed the interaction between IWS1 and LEDGF/p75 using various experimental approaches including NMR, ITC, AlphaScreen and pull-down assays. Moreover we showed that HIV-1 integrase, JPO2, PogZ and MLL1 can compete with IWS1-LEDGF/p75 interaction. However, we did not see extensive co-localization of LEDGF/p75 and IWS1 using confocal microscopy. In contrast to JPO2 and HIV integrase, knockdown of LEDGF/p75 also did not alter the IWS1 nuclear distribution. These results indicate that in contrast to integrase and JPO2, other nuclear determinants are dominant over LEDGF/p75 for the nuclear localization of IWS1. In this regard it is known that IWS1 interacts with the CTD of the large subunit of RNAPII complex through Spt6 (ref. 43 ). During the reviewing process of this manuscript, Gérard et al . published an independent study, which confirmed the existence of a LEDGF/p75-IWS1-Spt6 triple complex that was suggested to have an important function during HIV latency [46] . The existence of this complex was confirmed in our study. When HIV enters the cell, integrase must compete with cellular binding partners to interact with LEDGF/p75. While the high affinity of HIV IN for LEDGF/p75 has been documented previously [44] , our data provide a structure-based explanation. In comparison with the cellular partners, binding to HIV IN buries a considerably larger hydrophobic surface area. In addition to increased solvent exclusion and concomitant larger entropy gain, this larger interface also allows for additional electrostatic and van der Waals interactions to be established. In addition, the binding site on IN is structurally prearranged, in contrast to the unstructured IBM. Detailed characterization of LEDGF/p75 interaction interfaces is important in light of efforts to develop novel inhibitors to target IBD interactions with MLL1-menin or HIV-1 IN (reviewed in ref. 61 and ref. 54 ). From our results, it is clear that potential inhibitors targeting the LEDGF/p75 IBD might disturb other physiological interactions. The cyclic peptide inhibitor CP65, for example, has been shown to disrupt the interactions of LEDGF/p75 with JPO2, MLL1 and HIV IN [14] , [62] . Although small cyclic peptides bind to the IBD and can inhibit HIV replication and leukaemic transformation in cell lines, their overexpression does not lead to any apparent toxicity. On the other hand, highly selective inhibitors of the HIV-1 IN-IBD interaction, such as LEDGINs [54] , were developed by targeting the binding partner (that is, HIV IN) rather than LEDGF/p75. However, this strategy might be challenging to apply to the interaction of LEDGF/p75 with MLL N -fusions because the target would be intrinsically unstructured. In conclusion, our results unambiguously define a common LEDGF/p75 interaction interface shared by JPO2, PogZ, MLL1, IWS1 and HIV IN, which is most likely used by other known LEDGF interaction partners (ASK and MLL2; Fig. 7 ). We demonstrate that this part of the IBD serves as a recognition interface for an intrinsically disordered consensus motif, whereby LEDGF/p75 can act as a chromatin tethering factor for its binding partners. Use of a single interface for several protein–protein interactions with intrinsically disordered regions is analogous to other transcription regulators such as the kinase-inducible domain interacting (KIX) domain [63] . HIV has evolved an alternative way to bind this recognition interface and usurp the elegant molecular tethering mechanism of LEDGF/p75 to achieve efficient integration. 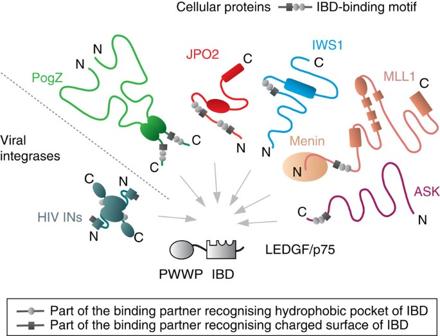Figure 7: Schematic representation of LEDGF/p75 IBD interactions. LEDGF/p75 uses a common specific region in the IBD for interactions with HIV IN and its cellular partners. Cellular binding partners interact with the IBD via an unstructured consensus motif. JPO2, PogZ and lentiviral integrase complexes can recruit more than one LEDGF/p75 molecule. Figure 7: Schematic representation of LEDGF/p75 IBD interactions. LEDGF/p75 uses a common specific region in the IBD for interactions with HIV IN and its cellular partners. Cellular binding partners interact with the IBD via an unstructured consensus motif. JPO2, PogZ and lentiviral integrase complexes can recruit more than one LEDGF/p75 molecule. Full size image Protein expression and purification Unlabelled IBD, PogZ 1117–1410 , IWS1 352–548 and JPO2 1–130 proteins were overexpressed from modified pMCSG7 vectors in E. coli BL21 (DE3) cells grown at 30 °C in lysogeny broth (LB) (Sigma) supplemented with 0.8% glycerol and 100 μg ml −1 ampicillin. When cultures reached an OD 550 nm of ∼ 0.8, heterologous expression was induced by addition of isopropyl-β-D-thiogalactopyranoside (IPTG). The IPTG concentration, duration and temperature of cultivation were optimized for individual proteins to achieve maximal protein yields. Optimal conditions were 0.25 mM IPTG, 5 h at 30 °C for JPO2; 0.2 mM IPTG, 4 h at 20 °C for the IBD; 0.25 mM IPTG, 4 h at 30 °C for PogZ 1117–1410 and 0.2 mM IPTG, 4 h at 30 °C for IWS1 352–548 . Bacterial cells were collected by centrifugation and resuspended in lysis buffer. The lysis buffer for the IBD, IWS1 352–548 and PogZ 1117–1410 was 25 mM sodium phosphate, pH 7.8, 1 M NaCl, 40 mM imidazole and 0.05% BME. For lysis of JPO2 1–130 , buffer containing 25 mM sodium phosphate, pH 8.0, 1 M NaCl, 15 mM imidazole and 0.05% BME was used. EDTA-free cOmplete protease inhibitor cocktail (Roche) tablets were added to the cell suspensions to block protease activity. Bacterial cells were disrupted by three passages through an Emulsiflex cell disrupter at 30 ksi. The lysate was centrifuged to remove insoluble materials, and the supernatant was used for further purification steps. The supernatant was clarified by filtration through a sterile Millex filter unit (porosity 0.8 μm; Millipore) and subjected to affinity chromatography using a HisTrap HP 5 ml column (GE Healthcare) equilibrated with lysis buffer. The His 6 -tagged protein was eluted in a gradient of lysis buffer supplemented with 400 mM imidazole, which was then eliminated from the sample by dialysis against lysis buffer without imidazole. The samples were incubated overnight with recombinant His 6 -tagged tobacco etch virus (TEV) protease at 16 °C to remove the affinity tag. Following TEV cleavage, a second round of His-Select Nickel Affinity Gel affinity chromatography was performed to remove TEV protease and uncleaved His 6 -tagged protein. The sample was then concentrated using Amicon Ultra Concentrators (Millipore). The final purification step was SEC on a Superdex 200 10/300 GL column using an Äkta Basic FPLC system (Amersham Biosciences) equilibrated in lysis buffer without imidazole. This purification protocol yielded 16.5 mg of purified IBD and 7.1 mg of purified PogZ 1117–1410 per liter of bacterial culture. The final yields of purified JPO2 1–130 and IWS1 352–548 were 5.1 and 9 mg, respectively, per liter of bacterial culture. The identities of purified JPO2 1–130 and IWS1 352–548 were confirmed by intact mass measurements (MALDI-TOF) and peptide mass fingerprinting (LC–MS), as there were irregularities in their gel migration behaviour typical for unstructured proteins ( Supplementary Fig. 9 ). Flag-tagged LEDGF/p75 and mutants were expressed and purified in the same way as described for non-tagged LEDGF/p75 (ref. 30 ). Production of wild-type (WT) MBP-JPO2 (ref. 45 ), MBP-PogZ 1117–1410 (ref. 31 ) and mutants thereof were performed as described earlier. GST-tagged LEDGF/p75, LEDGF/p52, PWWP, IBD, GST-LEDGF/p75 325–530 and GST-tagged Spt6 194–230 were expressed in E. coli BL21 grown on LB medium supplemented with 20 μg ml −1 ampicillin. Bacterial cultures were grown at 37 °C. Protein expression was induced with 1 mM IPTG at an OD 600 nm of 0.6. Cultures were harvested after 4 h. Pellets were washed in 20 ml STE buffer (10 mM Tris-HCl, pH 7.3, 100 mM NaCl, 0.1 mM EDTA), and stored at −20 °C. Cells were lysed in buffer containing 50 mM Tris-HCl, pH 7.5, 250 mM NaCl, 1 mM dithiothreitol (DTT), 0.1 μg ml −1 DNAse (Thermo Scientific) and protease inhibitor (cOmplete, EDTA-free, Roche). Purification was carried out by affinity chromatography on Glutathione Sepharose-4 Fast Flow (GE Healthcare, Fairfield, CT, USA). The resin was equilibrated with wash buffer (50 mM Tris-HCl, pH 7.5, 250 mM NaCl, 1 mM DTT), and GST-tagged proteins were eluted in wash buffer supplemented with 20 mM glutathione. The fractions were analysed by sodium dodecyl sulfate-polyacrylamide gel electrophoresis (SDS-PAGE) for protein content. Peak fractions were pooled and dialysed against 50 mM Tris-HCl, pH 7.5, 250 mM NaCl and 10% (v/v) glycerol. Full-length His-IWS1 was expressed in E. coli BL21 (DE3) at 30 °C. Protein expression was induced with 0.2 mM IPTG at an OD 600 nm of 0.8, and the culture was harvested after 3 h. Cells were washed in 20 ml STE buffer (10 mM Tris-HCl, pH 7.5, 100 mM NaCl, 0.1 mM EDTA). Cell pellets were resuspended in lysis buffer (50 mM Tris-HCl, pH 7.5; 150 mM NaCl, 20 mM imidazole, 0.1 μg ml −1 DNAse (Thermo Scientific) and protease inhibitor (cOmplete, EDTA-free, Roche)) and lysed by sonication. The lysate was cleared by centrifugation at 19,800 g for 30 min at 4 °C and subjected to affinity chromatography using His-Select Nickel Affinity Gel (Sigma) equilibrated with wash buffer (50 mM Tris-HCl, pH 7.5, 150 mM NaCl, 20 mM imidazole). His-tagged proteins were eluted with wash buffer containing 250 mM imidazole. Fractions were analysed by SDS-PAGE for protein content. Peak fractions were dialyzed against a 100-fold excess of 20 mM Tris-HCl, pH 7.5, 150 mM NaCl, 10% (v/v) glycerol at 4 °C overnight. Uniformly 15 N- and 15 N/ 13 C-labelled IBD, PogZ 1117–1410 and JPO2 1–130 were produced from cells grown in minimal media containing 15 N-ammonium sulfate and 13 C- D -glucose as the sole nitrogen and carbon sources. The media were supplemented with 20 μg ml −1 ampicillin, and cells were grown at 30 °C for 6 h before being transferred to 20 °C. After temperature stabilization, heterologous expression was induced by addition of IPTG. The final concentration of IPTG for both IBD and JPO2 1–130 expression was 0.2 mM with cultivation for 15 h at 20 °C; for PogZ 1117–1410 we used 0.2 mM IPTG, 16 h at 20 °C and for IWS1 352–548 0.2 mM IPTG, 14 h at 18 °C. The purification protocol for labelled proteins was the same as for the corresponding recombinant protein fragments expressed by cells grown in LB medium. CD spectroscopy Far-ultraviolet CD spectroscopy experiments were carried out using a Jasco 815 spectrometer at 20 °C. The buffer contained 10 mM sodium phosphate, pH 8.0, and 100 mM NaCl, with final protein concentrations of 0.125 mg ml −1 . The CD spectra were recorded from 190 to 300 nm in a 0.1 cm quartz cell. After baseline correction, the spectra were converted to molar ellipticity θ (deg cm 2 dmol −1 ) per residue, and the α-helical fractions were calculated. Analytical SEC Analytical SEC was performed using the Äkta Basic FPLC system (Amersham Biosciences) on a Superdex 200 10/300 GL Tricorn column (Pharmacia). The column was equilibrated with buffer containing 50 mM Tris-HCl, pH 7.8, 150 mM NaCl and 0.05% β-mercaptoethanol. The protein standards (Sigma-Aldrich) used for molecular weight estimation were blue dextran (2,000 kDa), bovine serum albumin (66 kDa), carbonic anhydrase (29 kDa), cytochrome c (12.4 kDa) and aprotinin (6.5 kDa). Differential scanning fluorimetry DSF analysis using a real-time PCR LightCycler 480 II (Roche) was performed to assess the stabilizing effects of various buffers and their effects on complex formation. Sixteen buffers (100 mM) covering the near neutral pH range were tested in the presence or absence of 200 mM NaCl as described by Ericsson et al . [64] . Proteins (0.1 mg ml −1 ) were assayed in the presence of 8 × Sypro Orange dye (Invitrogen) in a total reaction volume of 25 μl. The plates were sealed with LightCycler 480 Sealing Foil (Roche), and a temperature gradient from 20 to 95 °C with a rate of 1 °C min −1 was applied. The fluorescence intensity of Sypro Orange was recorded at 580 nm, with an excitation wavelength of 465 nm. All experiments were performed at least in duplicate. Isothermal titration calorimetry ITC experiments were performed using a MicroCal Auto-iTC200 System (GE Healthcare) at 25 °C. The samples were prepared in 50 mM Tris-HCl, pH 7.8, 150 mM NaCl, 0.05% BME. Protein concentrations were determined by amino-acid analysis. For the IBD-JPO2 1–130 complex, 2 μl aliquots of 60 μM JPO2 1–130 were injected stepwise into a sample cell containing 200 μl of 10 μM IBD. For the IBD-PogZ 1117–1410 complex, 2 μl aliquots of 114 μM PogZ 1117–1410 were injected stepwise into a sample cell containing 200 μl of 10 μM IBD. The samples for IWS1 titration experiments were prepared in 50 mM Tris-HCl, pH 8.5, 150 mM NaCl, 0.05% BME. For the IBD-IWS1 352–548 complex, 2 μl aliquots of 145 μM IWS1 352–548 were injected stepwise into a sample cell containing 200 μl of 15 μM IBD. Each assay was accompanied by a control experiment in which the binding buffer was titrated with the injected protein alone. All experiments were performed at least in triplicate. The association constants and stoichiometry ( N ) were estimated using MicroCal Origin software (GE Healthcare). Known variances of each measurement were used to calculate the weighted average of the dissociation constant ( K d ) and stoichiometry as a maximum likelihood estimator. NMR spectroscopy NMR spectra were acquired at 25 °C on a 600 MHz Bruker Avance spectrometer equipped with triple-resonance ( 15 N/ 13 C/ 1 H) cryoprobe. The sample volume was 0.35 ml, with protein concentrations ranging from 0.1 mM to 0.35 mM for free JPO2 1–130 , IBD, IWS1 352–548 and PogZ 1117–1410 proteins as well as IBD-JPO2 1–130 , IBD-IWS1 352–548 and IBD-PogZ 1117–1410 complexes in 25 mM HEPES, pH 7.0, containing 100 mM NaCl, 0.05% BME, 5% D 2 O/95% H 2 O. A series of double- and triple-resonance spectra were recorded to determine essentially complete sequence-specific resonance backbone assignments for the free IBD and backbone and side-chain assignments for the PogZ 1389–1404 bound IBD, as previously described [65] , [66] . The specific interactions of PogZ 1117–1410 , IWS1 352–548 or JPO2 1–130 with IBD were monitored by changes in the positions of signals of 15 N/ 13 C-labelled IBD in 3D HNCO spectra. From these changes, the most affected amino-acid residues were determined using the minimal backbone chemical shift ( 15 N, 13 C′ and 1 H N ) approach [67] . Amino-acid residues within these regions that were perturbed at least 1.5-fold the s.d. were then mapped on the structure of the IBD in complex with HIV IN (PDB ID 2B4J [38] ). The assignments for the bound PogZ 1389–1404 peptide were obtained using 13 C/ 15 N filtered homonuclear total correlation spectroscopy and NOESY experiments. 1 H– 1 H distance constraints required to calculate the structure of the IBD-PogZ 1389–1404 complex were derived from 3D 15 N/ 1 H NOESY-HSQC, 13 C/ 1 H HSQC-NOESY and in 2D 13 C/ 15 N-filtered/edited NOESY spectra, which were acquired using NOE mixing time of 120 ms. The family of converged structures for the IBD-PogZ 1389–1404 complex was initially calculated using Cyana 2.1. The combined automated NOE assignment and structure determination protocol [68] was used to automatically assign the NOE cross-peaks identified in NOESY spectra and to produce preliminary structures. In addition, backbone torsion angle constraints, generated from assigned chemical shifts using the program TALOS+ [69] were included in the calculations. Subsequently, five cycles of simulated annealing combined with redundant dihedral angle constraints were used to produce the sets of converged structures with no significant restraint violations (distance and van der Waals violations <0.2 Å), which were further refined in explicit solvent in YASARA ( http://www.yasara.org/ ). Analysis and validation of the family of structures obtained was carried out using the programs Molmol, iCING and PyMol. Pull-down assays A 40 μl aliquot of 10 μM GST-LEDGF/p75, GST-LEDGF/p75 325–530 , GST-IBD, GST-PWWP or GST-LEDGF/p52 was mixed with 40 μl Glutathione Sepharose resin (GE Healthcare) pre-equilibrated with wash buffer (50 mM Tris-HCl, pH 7.3, 200 mM NaCl) and incubated for 2 h at 4 °C. The beads were then washed five times with 600 μl wash buffer. The presence of proteins bound to the resin was confirmed by SDS-PAGE ( Fig. 5d ). SupT1 cells (NIH: SupT1 from Dr James Hoxie) nuclear extracts were prepared as described by Cherepanov et al . [16] . The cells were washed with PBS, harvested and lysed with 700 μl lysis buffer (50 mM Tris/HCl, pH 7.3, 150 mM NaCl, 0.5% (v/v) Triton X-100, 10% glycerol, cOmplete protease inhibitor cocktail (Roche, Germany)) for 10 min on ice. The lysate was cleared by centrifugation to divide nuclear and cytosolic fraction. To isolate the nuclear extract, the pellet was resuspended in 50 mM Tris/HCl, pH 7.3, 400 mM NaCl, 0.5% (v/v) Triton X-100, 10% glycerol, cOmplete protease inhibitor cocktail (Roche, Germany) and incubated for 30 min on ice and subsequently cleared by centrifugation. Extracts were diluted with 50 mM Tris-HCl, pH 7.3, bringing the salt concentration down to 200 mM. The lysate (1 ml) was added to the GST-tagged proteins bound to Glutathione Sepharose and incubated for 3 h at 4 °C. The beads were collected by centrifugation (60 s, 340 g , 4 °C) and washed five times in 600 μl lysis buffer. Bound proteins were eluted with 50 μl SDS-PAGE loading buffer and analysed by western blotting for the presence of IWS1 using 1:5,000 anti-IWS1 polyclonal rabbit antibody (Cell Signaling Technology, 5681S). Uncropped and marked scans of western blot and SDS-PAGE gel are available in Supplementary information ( Supplementary Fig. 10 ). AlphaScreen AlphaScreen measurements were performed in a total volume of 25 μl in 384-well Optiwell microtiter plates (PerkinElmer). The optimal protein concentrations for each experiment were determined by cross-titration to avoid binding curve perturbation while still yielding a high signal-to-noise ratio. All components were diluted in assay buffer (25 mM Tris-HCl, pH 7.4, 150 mM NaCl, 1 mM DTT, 0.1% (v/v) Tween-20 and 0.1% (w/v) bovine serum albumin). For binding curve determinations, MBP-JPO2 and MBP-PogZ 1117–1410 WT and/or mutants were titrated against 200 nM Flag-LEDGF/p75. For identification of the IWS1 interaction site on LEDGF, GST-LEDGF/p75, GST-LEDGF/p52, GST-PWWP, GST-LEDGF/p75 325–530 and GST-IBD were titrated against 20 nM His-IWS1. To assess the interaction effects of LEDGF/p75 mutants, WT or mutant LEDGF/p75 was titrated against 20 nM His-HIV-1 IN or His-IWS1 or 1 nM MPB-PogZ or MBP-JPO2. Plates were incubated for 1 h at 4 °C. Subsequently, a mix of AlphaScreen donor and acceptor beads (PerkinElmer) was added (final concentration 20 μg ml −1 ), bringing all proteins to the indicated final concentrations. After 1 h of incubation at 20 °C, the plate was analysed in an EnVision Multi-label Reader in AlphaScreen mode (PerkinElmer). Each titration was performed in duplicate, and assays were independently repeated three times. Results were analysed in Prism 5.0 (GraphPad software) after non-linear regression with the appropriate equations. One-site specific binding, taking ligand depletion into account, was used for the apparent K d measurements. Accession codes: The structures and assigned chemical shifts for the IBD-PogZ 1389–1404 complex were deposited in PDB and BMRB databases under accession codes 2n3a and 25639 , respectively. How to cite this article: Tesina, P. et al . Multiple cellular proteins interact with LEDGF/p75 through a conserved unstructured consensus motif. Nat. Commun. 6:7968 doi: 10.1038/ncomms8968 (2015).